PPARγ is an E3 ligase that induces the degradation of NFκB/p65 Nuclear factor-κB (NFκB) and peroxisome proliferator activated receptor-γ (PPARγ) are both transcription factors that perform distinct but overlapping roles in cellular regulation. Here we report that PPARγ acts as an E3 ubiquitin ligase, physically interacting with p65 to induce its ubiquitination and degradation. The ligand-binding domain of PPARγ interacts with the Rel Homology Domain region of NFκB/p65 to undergo robust ubiquitination and degradation that was independent of PPARγ transcriptional activity. Moreover, the ligand-binding domain of PPARγ delivered Lys48-linked polyubiquitin, resulting in the ubiquitination and degradation of p65. Lys28 was found to be critically important for PPARγ-mediated ubiquitination and degradation of p65, as it terminated both NFκB/p65-mediated pro-inflammatory responses and xenograft tumours. These findings demonstrate that PPARγ E3 ubiquitin ligase activity induces Lys48-linked ubiquitination and degradation of p65, and that this function is critical to terminate NFκB signalling pathway-elicited inflammation and cancer. Nuclear factor-κB (NFκB) is pivotal in cellular homoeostasis and immunoregulation. Activation of the NFκB pathway depends on stability of the inhibitor, IκBα [1] , [2] , [3] . However, NFκB activation can also be terminated in the absence of IκBα [4] , suggesting the existence of additional regulatory mechanisms. p65/RelA is regulated by ubiquitin- and proteasome-dependent degradation signals that terminate NFκB activation [5] , [6] . Transcriptional control of the vast majority of genes involved in inflammation requires NFκB activation, and evidence indicate that some E3 ubiquitin ligases appear to be essential for control of nuclear NFκB p65 by inducing its degradation [5] , [7] , [8] . Even though peroxisome proliferator activated receptor-γ (PPARγ) has a central role in adipocyte differentiation and glucose homeostasis [9] , [10] , it has been implicated in the pathology of numerous diseases including cancer [11] , [12] and can repress pro-inflammatory genes via trans-repression and transcriptional squelching [13] , [14] . Other studies have shown that PPARγ interacts with p65 to facilitate its nuclear export in response to bacterial stimuli [15] , and to inhibit NFκB transcriptional activity [16] , [17] , however, the molecular mechanism by which this occurs is still unclear. In this study, we found that PPARγ is an E3 ubiquitin ligase that targeted NFκB/65 to terminate NFκB activation by inducing p65 proteasome-dependent degradation. PPARγ induces p65 proteasome-dependent degradation Although PPARγ is a nuclear receptor, it is also constitutively present in the cytoplasm and nucleus [18] , [19] in human colonic HT29 cells ( Fig. 1a and Supplementary Fig. S1 ). However, in PPARγ −/− mouse embryonic fibroblast (MEF) or in PPARγ short hairpin RNA (shRNA)-silenced HT29 cells (expresses high levels of endogenous PPARγ compared with HEK293T cells), p65 protein levels were significantly increased ( Fig. 1b ). To investigate the regulation of p65 expression under steady-state conditions, we incubated PPARγ −/− MEF and PPARγ shRNA-silenced HT29 cells with cycloheximide to inhibit protein synthesis and observed a rapid decrease in p65 protein half-life ( Fig. 1d ). These results suggest that PPARγ significantly decreased the half-life of the p65 protein. Importantly, overexpressing PPARγ significantly induced the degradation of p65 in the nucleus and cytoplasm ( Fig. 1f ) without affecting p65 messenger RNA expression ( Fig. 1g and Supplementary Fig. S2a,b ) that was inhibited with the proteasome inhibitor MG132 ( Fig. 1h ), which is consistent with PPARγ significantly decreasing the half-life of the p65 protein ( Fig. 1i ). These findings suggest that PPARγ-induced p65 degradation was involved in proteasome-dependent degradation. Moreover, NFκB luciferase and electrophoretic mobility shift assay analysis (EMSA) analysis showed that PPARγ significantly reduced NFκB activation ( Supplementary Fig. S3a ) and DNA binding ( Supplementary Fig. S3b ), which was associated with PPARγ-induced p65 protein degradation. In contrast, in PPARγ −/− MEF or in PPARγ shRNA-silenced HT29 cells stimulated with TNF-α, there was an increase in NFκB activation ( Supplementary Fig. S3c,d ). These results suggest that PPARγ inhibited NFκB activation by inducing p65 proteasome-dependent degradation. 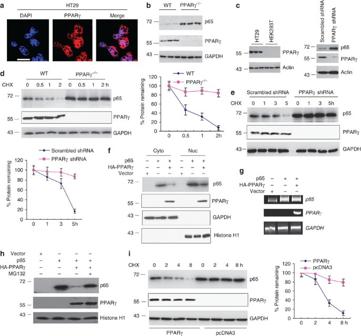Figure 1: PPARγ induces the degradation of p65. (a) Confocal immunofluorescence staining of PPARγ in HT29 cells. Scale bar, 30 μm. (b) Cell lysates from wild-type (WT) or PPARγ−/−MEF cells were subjected to western blotting as shown. (c) HT29 cells were transfected with scrambled shRNA or PPARγ shRNA for 36 h and cell lysates were subjected to western blotting. (d) WT or PPARγ−/−MEF cells were treated with cycloheximide (CHX, 30 μg ml−1) for 0, 0.5, 1 and 2 h to inhibitde novoprotein synthesis and harvested for western blotting. The levels of p65 at time 0 was set as 100% and the per cent p65 protein remaining following CHX treatment at each time point was calculated accordingly. (e) Control or PPARγ-silenced HT29 cells were treated with CHX (30 μg ml−1) for 0, 1, 3 and 5 h to inhibitde novoprotein synthesis and harvested for p65 western blotting. The per cent p65 protein remaining at each time point was calculated accordingly. (f,g) HEK293T cells were transfected with p65, HA-PPARγ or vector control for 36 h. Subcellular fractionations were subjected to western blotting (f) or RT-PCR analysis (g). (h) HEK293T cells were transfected with p65, HA-PPARγ or vector control for 36 h. Cells were treated with or without 10 μM MG132 for 6 h before cell lysis and subjected to western blotting as shown. (i) HEK293T cells were transfected with p65, HA-PPARγ or vector control. After 36 h, cells were treated with CHX (30 μg ml−1) for 0, 2, 4 and 8 h to inhibitde novoprotein synthesis and harvested for western blotting. The per cent p65 protein remaining at each time point was calculated accordingly. Data are triplicates from three independent experiments. DAPI, 4′,6-diamidino-2-phenylindole. Figure 1: PPARγ induces the degradation of p65. ( a ) Confocal immunofluorescence staining of PPARγ in HT29 cells. Scale bar, 30 μm. ( b ) Cell lysates from wild-type (WT) or PPARγ −/− MEF cells were subjected to western blotting as shown. ( c ) HT29 cells were transfected with scrambled shRNA or PPARγ shRNA for 36 h and cell lysates were subjected to western blotting. ( d ) WT or PPARγ −/− MEF cells were treated with cycloheximide (CHX, 30 μg ml −1 ) for 0, 0.5, 1 and 2 h to inhibit de novo protein synthesis and harvested for western blotting. The levels of p65 at time 0 was set as 100% and the per cent p65 protein remaining following CHX treatment at each time point was calculated accordingly. ( e ) Control or PPARγ-silenced HT29 cells were treated with CHX (30 μg ml −1 ) for 0, 1, 3 and 5 h to inhibit de novo protein synthesis and harvested for p65 western blotting. The per cent p65 protein remaining at each time point was calculated accordingly. ( f , g ) HEK293T cells were transfected with p65, HA-PPARγ or vector control for 36 h. Subcellular fractionations were subjected to western blotting ( f ) or RT-PCR analysis ( g ). ( h ) HEK293T cells were transfected with p65, HA-PPARγ or vector control for 36 h. Cells were treated with or without 10 μM MG132 for 6 h before cell lysis and subjected to western blotting as shown. ( i ) HEK293T cells were transfected with p65, HA-PPARγ or vector control. After 36 h, cells were treated with CHX (30 μg ml −1 ) for 0, 2, 4 and 8 h to inhibit de novo protein synthesis and harvested for western blotting. The per cent p65 protein remaining at each time point was calculated accordingly. Data are triplicates from three independent experiments. DAPI, 4′,6-diamidino-2-phenylindole. Full size image PPARγ interacts with p65 Under basal conditions, PPARγ is physically bound to p65 ( Fig. 2a ). However, PPARγ does not bind all the p65 protein and the remaining free p65 protein is relative stable ( Supplementary Fig. S4a ). This suggests that only the PPARγ that bound p65 induced its degradation. To quantify the physical relevance of the PPARγ/p65 complex in inducing p65 degradation, cells were treated with TNF-α or LPS to increase PPARγ binding to p65 ( Supplementary Fig. S4b ), which led to a rapid decrease in the half-life of the p65 protein ( Supplementary Fig. S4c ). The half-life of the p65 protein was about 15 min earlier as compared with unstimulated controls ( Fig. 1d ). The interaction of the PPARγ/p65 complex was confirmed by glutathione S-transferase (GST) pull-down assays that showed PPARγ was bound to p65 in the cytoplasm and the nucleus ( Fig. 2c ). Although PPARγ bound p65 and p50 ( Supplementary Fig. S5a,b ), PPARγ did not bind p50 in p65 −/− MEF cells ( Supplementary Fig. S5c ), suggesting that PPARγ indirectly bound to p50, as p50/p65 is a heterodimer. Thus, to determine the relative percentage of p65 that bound p50 and PPARγ, HEK293T cells were co-transfected with his-p65 together with Flag-PPARγ and Flag-p50. Ni-NTA pull-down analysis showed that p65 binding to PPARγ was about 50% higher than p50 ( Supplementary Fig. S5d ). IκBα interacts with p65 to inhibit nuclear translocation, and activation of IκB kinase can lead to the degradation of IκBα and translocation of p65 in the nucleus [1] , [2] . To determine whether IκBα can regulate PPARγ/p65 complex formation, cells were transfected with an IκBα superdominant (s.d.) stable mutant that lacks the IκB kinase phosphorylation sites [20] . Our results show that although IκBα was incorporated into the PPARγ/p65 complex, it did not affect PPARγ/p65 formation ( Supplementary Fig. S5e ). Moreover, p65 did not significantly bind PPARα or PPARβ ( Supplementary Fig. S6a ) or other NFκB components c-Rel, p52 or RelB ( Supplementary Fig. S6b ). PPARγ interaction with p65 was confirmed using Ni-NTA-Sepharose affinity chromatography, which demonstrated that PPARγ and p65 formed a complex ( Supplementary Fig. S7 ). Therefore, to determine the specific region(s) of p65 that interacted with PPARγ, we generated mutants of p65. As shown in Fig. 2d , PPARγ interacted with the Rel Homology Domain (RHD) fragments 19–306 but not with fragments 307–551 by GST pull-down analysis. Previous studies [21] have shown that the PPARγ ligand-binding domain (LBD) is important for activation so it was of interest to determine whether LBD could mediate the binding between PPARγ and p65. To address this, we used GST pull-down analysis which demonstrated that PPARγ significantly bound p65 whereas the PPARγ mutants lacking the LBD were unable to bind p65 ( Fig. 2e ). Similar results were observed by transfecting HEK293 cells with the LBD plasmid alone ( Supplementary Fig. S8 ). These results suggest that the LBD is critical for the interaction of PPARγ with p65. 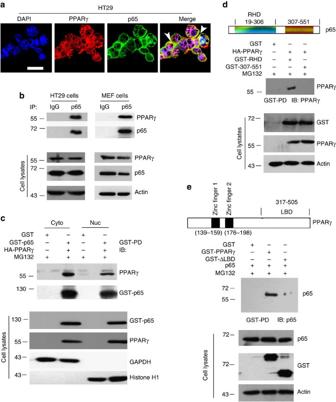Figure 2: PPARγ binds p65. (a) Confocal analysis of PPARγ interaction with p65 in HT29 cells. Arrow heads show PPARγ co-localized with p65. Scale bar, 30 μm. (b) HT29 or MEF cell lysates were subjected to immunoprecipitation and western blot analysis as shown. (c) HEK293T cells were transfected with GST-p65 and HA-PPARγ and subcellular fractions were subjected to GST pull-down (GST-PD) and western blotting. To inhibit protein degradation, cells were treated with 10 μM MG132 for 6 h before cell lysis. (d) Constructs of p65 (upper panel). Cell lysates of HA-PPARγ, GST-RHD or GST-307-551 transfected in HEK293T cells were subjected to GST pull-down and western blotting. Cells were treated with 10 μM MG132 for 6 h before cell lysis. (e) Constructs of PPARγ (upper panel). Cell lysates of p65, GST-PPARγ or GST-PPARγ-ΔLBD transfected in HEK293T cells were subjected to GST pull-down and western blotting. Cells were treated with 10 μM MG132 for 6 h before cell lysis. Data are triplicates from three independent experiments. DAPI, 4′,6-diamidino-2-phenylindole. Figure 2: PPARγ binds p65. ( a ) Confocal analysis of PPARγ interaction with p65 in HT29 cells. Arrow heads show PPARγ co-localized with p65. Scale bar, 30 μm. ( b ) HT29 or MEF cell lysates were subjected to immunoprecipitation and western blot analysis as shown. ( c ) HEK293T cells were transfected with GST-p65 and HA-PPARγ and subcellular fractions were subjected to GST pull-down (GST-PD) and western blotting. To inhibit protein degradation, cells were treated with 10 μM MG132 for 6 h before cell lysis. ( d ) Constructs of p65 (upper panel). Cell lysates of HA-PPARγ, GST-RHD or GST-307-551 transfected in HEK293T cells were subjected to GST pull-down and western blotting. Cells were treated with 10 μM MG132 for 6 h before cell lysis. ( e ) Constructs of PPARγ (upper panel). Cell lysates of p65, GST-PPARγ or GST-PPARγ-ΔLBD transfected in HEK293T cells were subjected to GST pull-down and western blotting. Cells were treated with 10 μM MG132 for 6 h before cell lysis. Data are triplicates from three independent experiments. DAPI, 4′,6-diamidino-2-phenylindole. Full size image PPARγ induces the ubiquitination of p65 As NFκB activation can be terminated by ubiquitin/proteasome-dependent degradation [4] , we determined whether PPARγ could induce the ubiquitination of p65. Our data reveal that PPARγ could significantly induce the ubiquitination of p65 ( Fig. 3a and Supplementary Fig. S9a ) in the RHD but not with the 307–551 fragments ( Supplementary Fig. S9b ). As predicted, silencing PPARγ in HT29 cells significantly decreased the ubiquitination of p65 ( Fig. 3b and Supplementary Fig. S9c ). Thus, to determine the physical function of PPARγ, PPARγ −/− MEF cells were reconstituted with PPARγ, C139A or C193A mutant, which significantly induced the ubiquitination of p65 in reconstituted PPARγ and C193A but not in PPARγ −/− or C139A mutant MEF cells ( Fig. 3c and Supplementary Fig. S10 ). Several RING finger domains function as E3 ligases to target substrate protein and to induce degradation by the proteasome pathway [22] , [23] . Although alignment analysis depicts a RING domain between the two zinc-finger domains of PPARγ ( Supplementary Fig. S11 ), it is still not clear whether PPARγ is an E3 ligase. As E3 ligase can develop polyubiquitin without substrate [22] , [23] , we established an in vitro ubiquitination analysis for PPARγ ligase activity using bacterially expressed recombinant human PPARγ along with different E2 (UBCH3, UBCH5a, b, c) in reaction buffer as described in experimental procedures. Our results revealed that UBCH3 but not UBCH5a/b/c was critical for PPARγ-mediated polyubiquitin formation ( Fig. 3d ). In addition, even though PPARγ could significantly induce polyubiquitin formation, the C139A mutant could not ( Fig. 3e ), and is in agreement with the findings that C139A/PPARγ could not induce the ubiquitination of p65 ( Fig. 3c ). Moreover, our studies show that purified PPARγ bound recombinant p65 directly ( Fig. 3f ) and significantly induced the ubiquitination of p65 whereas the C139A mutant in the zinc-finger domains did not ( Fig. 3g ). 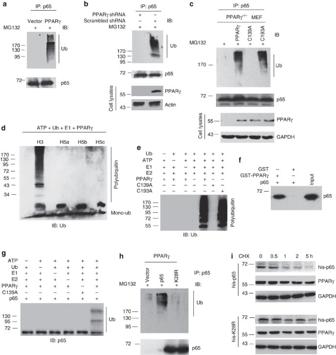Figure 3: PPARγ functions as an E3 ligase to induce the ubiquitination of p65. (a) HEK293T cells were transiently transfected with PPARγ for 36 h. Cell lysates were subjected to denatured immunoprecipitation and western blotting. Cells were treated with 10 μM MG132 for 6 h before cell lysis. (b) HT29 cells were transfected with scrambled shRNA or PPARγ shRNA for 36 h. Cell lysates were then subjected to denatured immunoprecipitation western blotting. Cells were treated with 10 μM MG132 for 6 h before cell lysis. (c) PPARγ−/−MEF cells or PPARγ−/−MEF cells were transiently transfected with PPARγ, C139A or C193A separately. Cell lysates were subjected to denatured immunoprecipitation and western blotting. Cells were treated with 10 μM MG132 for 6 h before cell lysis. (d)In vitropolyubiquitin formation analysis was performed (see experimental procedures) in reaction buffer contained different E2 (UBCH3, UBCH5a, b, c) with 10ng PPARγ or (e) containing UBCH3 with 10 ng PPARγ, C139A or C193A as indicated. Reactions were incubated at 30 °C for 2 h. The ubiquitinated products were detected with an ubiquitin antibody. (f) GST pull-down assay in which GST-PPARγ or GST alone bound to glutathione-agarose beads was incubated with recombinant p65. (g)In vitroubiquitination of p65 analysis was performed (see experimental procedures) in the reaction buffer contained UBCH3, p65 (10 μg) and 10 ng PPARγ (WT or C139A) as indicated. Reactions were incubated at 30 °C for 2 h, resolved by SDS–PAGE and the ubiquitinated products were detected with p65 antibody. (h) HEK293 cells were transfected with PPARγ, his-p65 or K28R. Cell lysates were subjected to denatured Ni-NTA pull-down and western blotted. Cells were treated with 10 μM MG132 for 6 h before cell lysis. (i) HT29 cells were transfected with his-p65 or his-p65/K28R plasmids and after 36 h, cells were treated with cycloheximide (30 μg ml−1) for 0, 0.5, 1, 2 and 5 h to inhibitde novoprotein synthesis and harvested for p65 by western blot. Data are triplicates from three independent experiments. Figure 3: PPARγ functions as an E3 ligase to induce the ubiquitination of p65. ( a ) HEK293T cells were transiently transfected with PPARγ for 36 h. Cell lysates were subjected to denatured immunoprecipitation and western blotting. Cells were treated with 10 μM MG132 for 6 h before cell lysis. ( b ) HT29 cells were transfected with scrambled shRNA or PPARγ shRNA for 36 h. Cell lysates were then subjected to denatured immunoprecipitation western blotting. Cells were treated with 10 μM MG132 for 6 h before cell lysis. ( c ) PPARγ −/− MEF cells or PPARγ −/− MEF cells were transiently transfected with PPARγ, C139A or C193A separately. Cell lysates were subjected to denatured immunoprecipitation and western blotting. Cells were treated with 10 μM MG132 for 6 h before cell lysis. ( d ) In vitro polyubiquitin formation analysis was performed (see experimental procedures) in reaction buffer contained different E2 (UBCH3, UBCH5a, b, c) with 10ng PPARγ or ( e ) containing UBCH3 with 10 ng PPARγ, C139A or C193A as indicated. Reactions were incubated at 30 °C for 2 h. The ubiquitinated products were detected with an ubiquitin antibody. ( f ) GST pull-down assay in which GST-PPARγ or GST alone bound to glutathione-agarose beads was incubated with recombinant p65. ( g ) In vitro ubiquitination of p65 analysis was performed (see experimental procedures) in the reaction buffer contained UBCH3, p65 (10 μg) and 10 ng PPARγ (WT or C139A) as indicated. Reactions were incubated at 30 °C for 2 h, resolved by SDS–PAGE and the ubiquitinated products were detected with p65 antibody. ( h ) HEK293 cells were transfected with PPARγ, his-p65 or K28R. Cell lysates were subjected to denatured Ni-NTA pull-down and western blotted. Cells were treated with 10 μM MG132 for 6 h before cell lysis. ( i ) HT29 cells were transfected with his-p65 or his-p65/K28R plasmids and after 36 h, cells were treated with cycloheximide (30 μg ml −1 ) for 0, 0.5, 1, 2 and 5 h to inhibit de novo protein synthesis and harvested for p65 by western blot. Data are triplicates from three independent experiments. Full size image Several lines of evidence demonstrate that although Lys(K)63 linked target proteins for ubiquitination, K48-linked target proteins are destined for proteasomal-mediated degradation [24] . Moreover, recent studies [25] have shown that in addition to K48, the K6, K11, K27, K29 and K33-linked polyubiquitin chains are also involved in proteasomal degradation. Even though we demonstrated that PPARγ functions as an E3 ligase to induce the ubiquitination of p65, it was still not clear which lysine-linked polyubiquitin targeted the p65 protein. To address this, in vivo ubiquitinated forms of N-terminal GST-fused p65 protein in response to PPARγ were purified and analysed by liquid chromatography coupled with tandem mass spectrometry (LC/MS/MS). Our results show that PPARγ induced K48-linked polyubiquitination of p65 ( Fig. 4a ) that was confirmed using a K48 mutant ( Fig. 4b ), suggesting that K48-linked polyubiquitin was critically important for PPARγ-mediated regulation of p65. As PPARγ could significantly induce the ubiquitination of p65 in the RHD, it was of interest to identify the K48 polyubiquitin target lysine residue in the RHD ( Fig. 4c ). To do this, lysine residues were replaced with arginine and the mutant plasmids co-transfected with PPARγ into HEK293T cells. Western blot analysis and NFκB luciferase assay showed that Lys28R of p65 significantly decreased PPARγ-mediated p65 degradation ( Fig. 4d ) and NFκB activation ( Fig. 4e ), suggesting that polyubiquitin targeted to Lys28 of p65 in response to PPARγ resulted in the ubiquitination and degradation of p65. These results are consistent with the findings that PPARγ could not induce the ubiquitination of p65/K28 ( Fig. 3h ) or reduce the half-life of the p65/K28 protein in HT29 cells overexpressing p65/K28R ( Fig. 3i ). 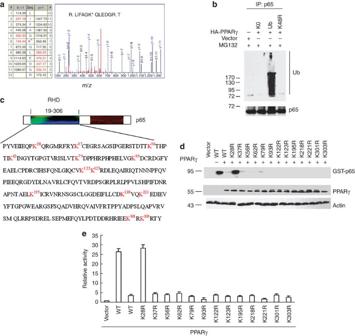Figure 4: Lys28 is required for PPARγ-mediated p65 degradation. (a) HEK293T cells were transfected with GST-p65 and PPARγ, and cell lysates were subjected to GST pull-down and SDS–PAGE. The Coomassie-stained proteins were excised and subjected to LC/MS/MS analysis. One of seven lysine residues of ubiquitin produces an isopeptide linkage with the C-terminus of another ubiqutin moiety, forming ubiquitin chains of various lengths and shapes (Lys 6, Lys 11, Lys 27, Lys 29, Lys 33 and Lys 63), but trypsin cannot cleave Gly–Gly modified lysine, therefore, ubiquitinated peptides are identified by a 114.1 Da diglycine (GG) tag on lysine residues, which is derived from the C-terminus of ubiquitin by trypsin cleavage. The full tryptic peptide LIFAGK*QLEDGR with K48 modified by GG is shown. K* depicts the lysine residue modified by isopeptide linkages. (b) HEK293T cells were transfected with HA-PPARγ, HA-ubiquitin (Ub) or HA-ubiquitin mutant (K0 or K48R) plasmids. Cell lysates were subjected to denatured immunoprecipitation and western blotting. Cells were treated with 10 μM MG132 for 6 h before cell lysis. (c) A schematic representation of the lysine mutants of p65/RHD used in this study (upper panel). (d) HEK293T cells were transfected with HA-PPARγ, GST-p65 or with the K→R mutant plasmids. Cell lysates were subjected to western blotting. (e) NFκB promoter activity in HA-PPARγ, p65 or the K→R mutants transfected in HEK293T cells. Results are expressed as means±s.e.m. (n=3). Figure 4: Lys28 is required for PPARγ-mediated p65 degradation. ( a ) HEK293T cells were transfected with GST-p65 and PPARγ, and cell lysates were subjected to GST pull-down and SDS–PAGE. The Coomassie-stained proteins were excised and subjected to LC/MS/MS analysis. One of seven lysine residues of ubiquitin produces an isopeptide linkage with the C-terminus of another ubiqutin moiety, forming ubiquitin chains of various lengths and shapes (Lys 6, Lys 11, Lys 27, Lys 29, Lys 33 and Lys 63), but trypsin cannot cleave Gly–Gly modified lysine, therefore, ubiquitinated peptides are identified by a 114.1 Da diglycine (GG) tag on lysine residues, which is derived from the C-terminus of ubiquitin by trypsin cleavage. The full tryptic peptide LIFAGK*QLEDGR with K48 modified by GG is shown. K* depicts the lysine residue modified by isopeptide linkages. ( b ) HEK293T cells were transfected with HA-PPARγ, HA-ubiquitin (Ub) or HA-ubiquitin mutant (K0 or K48R) plasmids. Cell lysates were subjected to denatured immunoprecipitation and western blotting. Cells were treated with 10 μM MG132 for 6 h before cell lysis. ( c ) A schematic representation of the lysine mutants of p65/RHD used in this study (upper panel). ( d ) HEK293T cells were transfected with HA-PPARγ, GST-p65 or with the K→R mutant plasmids. Cell lysates were subjected to western blotting. ( e ) NFκB promoter activity in HA-PPARγ, p65 or the K→R mutants transfected in HEK293T cells. Results are expressed as means±s.e.m. ( n =3). Full size image PPARγ transcription does not induce p65 degradation To determine whether PPARγ-induced p65 degradation was independent of its transcriptional activity, we deleted the potential nuclear location signal (NLS; 184–189 amino acids, http://www.receptors.org/NR/NLS/NLS_index.html ). As predicted, overexpressed PPARγ was significantly translocated into the nucleus ( Fig. 5a top panel merged photomicrograph) whereas, in cells expressing the deleted NLS, PPARγ was retained in the cytoplasm ( Fig. 5a bottom panel) and had significantly decreased PPARγ transcriptional activity ( Fig. 5b ). Although the deleted NLS of PPARγ decreased transcriptional activity ( Fig. 5b ), the PPARγ-ΔNLS was still able to induce the ubiquitination and degradation of p65 ( Fig. 5c ). As expected, the C139A mutant of PPARγ had no effect on its transcriptional activity ( Fig. 5b ) and did not induce the ubiquitination ( Fig. 5c ) and degradation of p65 ( Fig. 5d ). These results show that PPARγ-induced p65 degradation was independent of its transcriptional activity and that the zinc-finger of PPARγ functions as an E3 ligase to induce the degradation of p65. 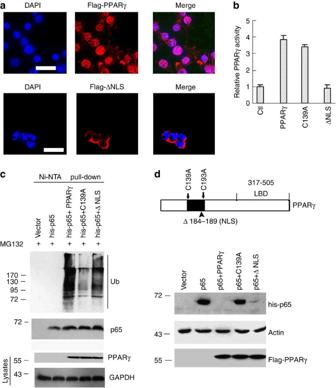Figure 5: PPARγ-induced p65 degradation is independent of its transcriptional activity. (a) HEK293 cells were transfected with Flag-PPARγ or Flag-PPARγ-ΔNLS and stained with Flag antibody and visualized by confocal microscopy. Scale bar, 30 μm. (b) HEK293T cells were transfected with PPRE3-luciferase reporter and PPARγ or mutant plasmids as indicated for 36 h, and PPARγ transcriptional activity were assayed. (c) HEK293T cells were transfected with the plasmids as indicated, and cell lysates were subjected to denatured Ni-NTA pull-down and western blotting. Cells were treated with 10 μM MG132 for 6 h before cell lysis. (d) Construct of PPARγ and mutant site (upper panel). HEK293T cells were transfected with the plasmids as indicated and cell lysates were subjected to western blotting. Figure 5: PPARγ-induced p65 degradation is independent of its transcriptional activity. ( a ) HEK293 cells were transfected with Flag-PPARγ or Flag-PPARγ-ΔNLS and stained with Flag antibody and visualized by confocal microscopy. Scale bar, 30 μm. ( b ) HEK293T cells were transfected with PPRE3-luciferase reporter and PPARγ or mutant plasmids as indicated for 36 h, and PPARγ transcriptional activity were assayed. ( c ) HEK293T cells were transfected with the plasmids as indicated, and cell lysates were subjected to denatured Ni-NTA pull-down and western blotting. Cells were treated with 10 μM MG132 for 6 h before cell lysis. ( d ) Construct of PPARγ and mutant site (upper panel). HEK293T cells were transfected with the plasmids as indicated and cell lysates were subjected to western blotting. Full size image PPARγ ligands increase PPARγ E3 ligase activity The studies above show that the LBD domain of PPARγ interacted with p65 ( Fig. 2e ). Thus, to determine whether the LBD domain of PPARγ is required for PPARγ-mediated p65 ubiquitination and degradation, we deleted the LBD domain. Truncating the LBD domain markedly decreased PPARγ-mediated ubiquitination of p65 ( Supplementary Fig. S12a,b ). Similarly, in the mutant LBD, PPARγ-mediated p65 degradation and DNA binding was significantly decreased ( Supplementary Fig. S12c,d ). These findings suggest that the LBD of PPARγ was required for binding p65 and to induce its degradation. As ligands of PPARγ can activate its function [21] , we next determine whether ligands of PPARγ can increase PPARγ E3 ligase function. As shown in Fig. 6a , activating PPARγ with troglitazone (TROG) or pioglitazone (PIOG) for 15 min significantly increased PPARγ binding to p65 and induced its ubiquitination. Moreover, cycloheximide chase assays showed that both TORG and PIOG can significantly decrease the half-life of the p65 protein ( Fig. 6c ). These results demonstrate that activating PPARγ can significantly increase the degradation of the p65 protein. 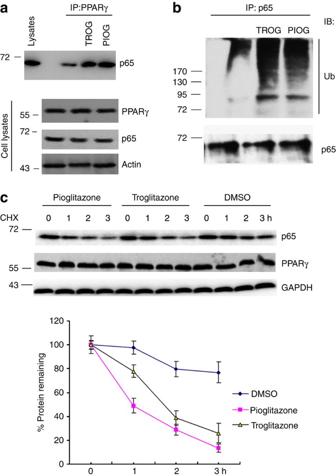Figure 6: Ligands of PPARγ increases PPARγ E3 activity. (a,b) HT29 cells were treated with 100 μM TROG or PIOG for 15 min and cell lysates were subjected to immunoprecipitation and western blotting as indicated. (c) HT29 cells were pretreated with TROG/PIOG for 15 min and then treated with cycloheximide (30 μg ml−1) for 0, 1, 2 and 3 h to inhibitde novoprotein synthesis and harvested for western blotting. The per cent p65 protein remaining at each time point was calculated accordingly. The carrier dimethylsulphoxide (DMSO) served as a control. Data are triplicates from three independent experiments. Figure 6: Ligands of PPARγ increases PPARγ E3 activity. ( a , b ) HT29 cells were treated with 100 μM TROG or PIOG for 15 min and cell lysates were subjected to immunoprecipitation and western blotting as indicated. ( c ) HT29 cells were pretreated with TROG/PIOG for 15 min and then treated with cycloheximide (30 μg ml −1 ) for 0, 1, 2 and 3 h to inhibit de novo protein synthesis and harvested for western blotting. The per cent p65 protein remaining at each time point was calculated accordingly. The carrier dimethylsulphoxide (DMSO) served as a control. Data are triplicates from three independent experiments. Full size image PPARγ inhibits NFκB/p65-mediated tumour growth Previous studies have shown that overexpressing p65 can lead to tumour growth [26] , so we next determine whether PPARγ can reduce p65-mediated tumour growth using a nude mice xenograft tumour model. As shown in Fig. 7a , PPARγ but not the C139A and K28R mutants significantly inhibited p65-induced tumour growth by reducing p65 protein levels. In addition, PPARγ −/− led to markedly increase tumour growth with a concomitant increase in p65 protein levels ( Fig. 7b and Supplementary Fig. S13a ). As PPARγ can induce the degradation of p65 and terminate NFκB transcriptional activity, we next determine if PPARγ can reduce NFκB/p65-mediated targeted gene expression. Real-time analysis showed that overexpressing p65 increased the expression of several genes that were significantly inhibited by PPARγ ( Supplementary Fig. S14 ). As C139 is the PPARγ E3 ligase activity site and K28 of p65 is the polyubiquitin-targeted site in response to PPARγ, we next investigated how PPARγ regulated NFκB/p65-mediated pro-inflammatory gene expression by real-time PCR analysis. Our results show that PPARγ but not the C139A mutant could significantly inhibit NFκB/p65-mediated pro-inflammatory Cox-2 and IL-1β gene expression, whereas the K28R mutant of p65 had no effect ( Fig. 7c–f ). Moreover, the PPARγ activator, PIOG, significantly inhibited tumour growth by reducing p65 protein levels ( Fig. 6g and Supplementary Fig. S13b ) and decreased pro-inflammatory Cox-2 and IL-1β gene expression in response to TNF-α ( Fig. 7h ). Taken together, these results suggest that PPARγ function as an ubiquitin ligase to terminate NFκB-mediated tumour growth and a schematic representation on how this occurs is shown in Fig. 8 . 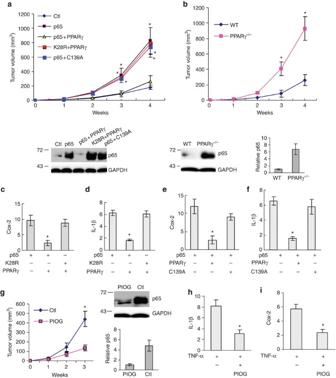Figure 7: PPARγ inhibits NFκB-mediated tumour growth. (a) Stable expressing plasmids in HT-29 cells (4 × 105) were injected subcutaneously in nude mice for 4 weeks, and tumour volume was measured. Results are expressed as means±s.e.m. (n=5; *P<0.05). p65 levels were determined from tumour lysates by western blotting (lower panel). (b) WT or PPARγ−/−MEF cells (4 × 105) were injected subcutaneously in nude mice and after 4 weeks tumour volume was measured and results are expressed as means±s.e.m. (n=5; *P<0.05). Tumour lysates were subjected to western blotting and p65 expression was quantitated. (c–f) HEK293T cells were transfected with the plasmids as indicated for 36 h, and Cox-2 or IL-1β gene expression were assayed by real-time PCR. *P<0.05. Results are expressed as means±s.e.m. (n=3). (g) HT-29 cells (1 × 106) were injected subcutaneously in nude mice and given PBS (Control, Ctl) or PIOG (20 mg kg−1per day) for 3 weeks by oral gavage. Tumour volume was then measured and results are expressed as means±s.e.m. (n=5; *P<0.05). Tumour lysates were subjected to western blotting and p65 expression was quantitated. (h,i) Mice were given PBS or PIOG for 3 days by oral gavage and then injected intravenously with 2 μg murine TNF-α for 6 h. Colonic tissues were collected, and Cox-2 and IL-1β gene expression were assayed by real-time PCR. *P<0.05. Results are expressed as means±s.e.m. (n=5). Figure 7: PPARγ inhibits NFκB-mediated tumour growth. ( a ) Stable expressing plasmids in HT-29 cells (4 × 10 5 ) were injected subcutaneously in nude mice for 4 weeks, and tumour volume was measured. Results are expressed as means±s.e.m. ( n =5; * P <0.05). p65 levels were determined from tumour lysates by western blotting (lower panel). ( b ) WT or PPARγ −/− MEF cells (4 × 10 5 ) were injected subcutaneously in nude mice and after 4 weeks tumour volume was measured and results are expressed as means±s.e.m. ( n =5; * P <0.05). Tumour lysates were subjected to western blotting and p65 expression was quantitated. ( c – f ) HEK293T cells were transfected with the plasmids as indicated for 36 h, and Cox-2 or IL-1β gene expression were assayed by real-time PCR. * P <0.05. Results are expressed as means±s.e.m. ( n =3). ( g ) HT-29 cells (1 × 10 6 ) were injected subcutaneously in nude mice and given PBS (Control, Ctl) or PIOG (20 mg kg −1 per day) for 3 weeks by oral gavage. Tumour volume was then measured and results are expressed as means±s.e.m. ( n =5; * P <0.05). Tumour lysates were subjected to western blotting and p65 expression was quantitated. ( h , i ) Mice were given PBS or PIOG for 3 days by oral gavage and then injected intravenously with 2 μg murine TNF-α for 6 h. Colonic tissues were collected, and Cox-2 and IL-1β gene expression were assayed by real-time PCR. * P <0.05. Results are expressed as means±s.e.m. ( n =5). 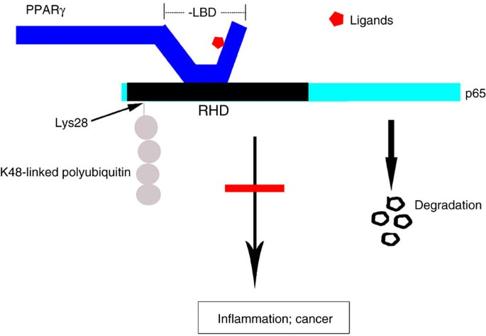Figure 8: A model depicting how PPARγ induces the degradation of p65. Ligands or agonists of PPARγ (for example, TROG, PIOG) induces PPARγ binding to p65, which subsequently transfers the K48-linked polyubiquitin to p65 promoting its degradation in a proteasome-dependent manner and abrogated NFκB/p65-mediated inflammation and cancer. Full size image Figure 8: A model depicting how PPARγ induces the degradation of p65. Ligands or agonists of PPARγ (for example, TROG, PIOG) induces PPARγ binding to p65, which subsequently transfers the K48-linked polyubiquitin to p65 promoting its degradation in a proteasome-dependent manner and abrogated NFκB/p65-mediated inflammation and cancer. Full size image IκBα-mediated nuclear export of the NFκB complex appears to be the central mechanism terminating NFκB signalling. In addition, both ubiquitin- and proteasome-dependent degradation of the NFκB p65 subunit are also important for efficient and prompt termination of NFκB activation [2] , [3] . The nuclear E3 ligases PDLIM2 and COMMD1 inhibit NFκB activation by inducing nuclear p65 degradation [5] , [6] , [22] , [27] , [28] . PPARγ can also repress pro-inflammatory genes by reducing NFκB transcriptional activity [16] , [17] , or can interact with active p65 and facilitate its nuclear export in response to bacterial stimuli, subsequently inhibiting NFκB activation [15] . Interestingly, here we found that PPARγ physically interacted with p65 in the cytoplasm and nucleus and significantly induced its degradation. These results suggest that PPARγ not only induced nuclear p65 degradation but also reduced cytoplasm p65 entering the nucleus by enhancing its degradation. Many RING finger domains simultaneously bind ubiquitination enzymes and their substrates and hence function as ligases. Ubiquitination in turn, targets the substrate protein for degradation [22] , [23] . HECT or RING/U-box domains are the major types of E3s in eukaryotes [22] , however, the E3 ligase, PDLIM2 with LIM domain, does not have these major domains [24] , suggesting some E3 ligases cannot be predicted by available methods. The zinc ligation topology of RING fingers is distinct and is referred to as a ‘cross-brace’ motif [22] ( Supplementary Fig. S11 ). In our studies, we found that the cooperation of two zinc-finger domains developed a RING domain ( Supplementary Fig. S11 ) that significantly induced polyubiquitination formation and in this process UBCH3 but not UBHC5a/b/c was critical for PPARγ-mediated polyubiquitination formation. These findings reveal a novel functional role for PPARγ as an E3 ubiquitin ligase. RING domains possess conserved Cys and His residues critical for E3 activity [22] , [23] as the residues of Y (number 3) and V (number 4) are not conserved C or H in loop 2 on PPARγ ( Supplementary Fig. S11 ). Thus, it was not surprising that the C139A but not the C193A mutant of PPARγ decreased its E3 ligase activity, suggesting that loop1 was critical for PPARγ E3 ligase activity. Moreover, even though PPARγ is a nuclear receptor, PPARγ-induced p65 degradation was independent of its transcriptional activity as the deleted NLS still induced the degradation of p65. Although the NLS is located inside the RING domain, the C-terminal portion of the ‘RING’ domain containing the NLS was not required for ubiquitination, as the C193A mutant did not affect PPARγ E3 ligase activity ( Fig. 3c/e ). These findings reinforce the notion that that loop1 but not loop2 on PPARγ has a critical role as an E3 ligase. PPARγ has a essential role in several diseases and thus, it is not surprising its expression is low in colon cancer patients and inhibitory when expression is high [29] . Similarly, colon tumours induced by carcinogens can be suppressed by PPARγ agonists, suggesting that PPARγ may act as a tumour suppressor [30] , [31] . Some important classes of synthetic agonists of PPARγ are TROG and PIOG, which can activate PPARγ by binding its LBD [17] , [32] . In our studies, we found that PPARγ agonists TROG and PIOG significantly induced PPARγ binding to p65 and led to the degradation p65 in vitro and in vivo . These findings unravel a novel function for PPARγ in inhibiting NFκB activation. NFκB seems to be a pivotal protein and a link between inflammation and cancer [33] . Deficiency in or hyper activation of NFκB results in inflammation [34] and is also a major hallmark of tumors [35] . Our findings show that PPARγ binds p65 and causes it to degrade effectively terminating NFκB hyper activation and provide novel evidence for PPARγ function as an inhibitor of inflammation and possibly cancer. Even though both E3 ligases (COMMD1 and PDLIM2) can induce the degradation of p65 (refs 5 , 23 ) [5] , [23] , they did not show any polyubiquitin-linked lysine site. Our studies revealed that lysine 28 residue of p65 was the critical polyubiquitin target site in response to PPARγ, as a mutant of lysine 28 (K28R) terminated PPARγ-induced p65 ubiquitination and degradation. Although evidence indicate that Lys63 linked target proteins for ubiquitination and Lys48 linked target proteins for proteasome-mediated degradation [24] , recent studies show that Lys6-, Lys11-, Lys27-, Lys29-, Lys33-, Lys48-linked polyubiquitin chains are also involved in proteasomal degradation [25] . Here we found that the Lys48-linked polyubiquitin chain targeted p65 by PPARγ ubiquitin ligase subsequently terminating p65 activation. These findings reveal that PPARγ function as a novel E3 ubiquitin ligase to induce Lys48-linked ubiquitination and degradation of p65, which is crucial for NFκB signalling in cancer and inflammation. Cell lines, plasmids and transfections The human colonic adenocarcinoma HT29 cells and MEF cells were obtained from the ATCC (Manassas, VA) and maintained in 10% fetal bovine serum (FBS) DMEM. HEK293T cells were maintained in 10% FBS DMEM medium. PPARγ −/− MEF cell lines were generous provided by Dr Spiegelman (Dana-Farber Cancer Institute). p65 −/− MEF cells were generous provided by Dr Hoffmann (University of California, San Diego). These cells were maintained in 10% FBS DMEM medium. The PPRE 3 -Lu plasmid was generous provided by Dr Stephen Safe (Institute of Biosciences and Technology, Texas A&M University). The PEBB-p65 plasmid was provided by Dr Burstei (UT Southwestern Medical Center at Dallas). HA-PPARγ cDNA was cloned into pcDNA3 vector, and PPARγ or p65 cDNA was cloned into PEBG vector. HA-IκBα s.d. has been described previously [20] . HA-PPARγ-ΔLBD, GST-PPARγ-ΔLBD, PEBB-p65-ΔRHD, GST-p65-Δ19-90, GST-Δ91-200, GST-Δ201-306, GST-p65-28R, GST-p65-37R, GST-p65-56R, GST- p65-62R, GST- p65-79R, GST- p65-93R, GST- p65-122R, GST-p65-123R, GST-p65-195R, GST-p65-218R, GST-p65-221R, GST-p65-301R, GST-p65-303R, HA-K6Ub, HA-K11Ub, HA-K27Ub, HA-K29Ub, HA-K33Ub, HA-K48Ub and HA-K63Ub were mutated by the QuickChange site-directed mutagenesis method, and all the plasmids were identified by DNA sequencing. PPARγ shRNA were obtained from Thermo Fisher Scientific. Plasmids were transfected by LipfectAMINE2000 according to the manufacturer’s instructions (Invitrogen). GST, PPARγ, p65, Flag and HA were from Delta Biolabs. Ubiquitin (P4D1), PPARα, PPARβ and p65 were from Santa Cruz. p52, c-Rel and RelB were from Cell Signaling Technology. Secondary antibodies were obtained from Jackson Immunoresearch. Immunofluorescence Cells were fixed for 15 min with 3.7% paraformaldehyde, incubated with primary antibodies and subsequently with secondary antibodies (Jackson Immunoresearch). After final washing, cells were covered with Permafluor mounting medium. Immunostained cells were viewed in a confocal microscope (OLYMPUS FV 1000 Confocal). Expression of recombinant protein Human PPARγ and p65 cDNA were cloned into PGEX-6P-1 vector and was identified by DNA sequencing. GST-PPARγ and GST-p65 were expressed in E. coli strain BL21(DE3) [pAPlacIQ]. The recombinant protein was purified using glutathione beads, and the GST-tags were removed by thrombin (Thermo Scientific). In vitro ubiquitination assay Polyubiquitination formation assay contained 50 mM Tris–HCl, pH 7.4, 10 mM MgCl 2 , ATP-regenerating system, 0.2 mM dithiothreitol, 50 μM ZnCl 2 , E1 (0.1 μM; Boston Biochem), E2 (UBCH3, UBCH5α/b,c, 0.4 μM), Ub (5 μg), 10 ng PPARγ (wild type (WT), C139A or C193A mutant). Reactions were incubated at 30 °C for 2 h and were terminated by EDTA (10 mM). Dithiothreitol (5 mM) was added into the reaction mixture at room temperature for 15 min to release ubiquitin from E1 and E2. The ubiquitinated products were detected by immunoblotting using an ubiquitin antibody. Ubiquitination of p65 assay contained 50 mM Tris–HCl, pH 7.4, 10 mM MgCl 2 , ATP-regenerating system, 0.2 mM dithiothreitol, 50 μM ZnCl 2 , E1 (0.1 μM; Boston Biochem), UBCH3 (0.4 μM), Ub (5 μg), p65 (10 μg), and 10 ng PPARγ (WT or C139A mutant). Reactions were incubated at 30 °C for 2 h, the ubiquitinated products were detected by immunoblotting with p65 antibody. Pull-down, western blot and LC/MS/MS analysis GST pull-down analysis was performed using the profound pull-down kit (Thermo Scientific). Cells were washed with ice-cold phosphate-buffered saline and lysed in detergent buffer [3] . Subcellular fractionation and immunoprecipitation was performed as described previously [3] . For denatured immunoprecipitation, cell extracts were heated at 95 °C for 5 min in the presence of 1% SDS to disrupt the non-covalent protein interactions. The SDS was diluted and the proteins were subjected to immunoprecipitation and western blotting. The samples were subjected to 10–20% gradient SDS–polyacrylamide gel electrophoresis (SDS–PAGE), transferred to a nitrocellulose membrane, then probed by western blot analysis with the indicated antibody and developed by using an ECL Kit (Amersham Biosciences). HEK293T cells were transfected with GST-p65 and PPARγ, cell lysates were subjected to GST pull-down, SDS–PAGE, Coomassie Brillant Blue stain, and the ubiquitinated p65 gel bands were excised and analysed by LC/MS/MS [36] at the Southern Alberta Mass Spectrometry Centre for Proteomics, a Core Facility at the University of Calgary; the MS-MS data were analysed using SwissProt data base search tool. Ni-NTA purification and pull-down For native Ni-NTA purification or pull-down, cells were washed with cold PBS and lysed in lysis buffer (50 mM NaH 2 PO4, 300 mM NaCl containing protease inhibitors (PMSF, Aprotinin, Leupeptin, E64), pH 8.0), sonicated and spun down. The supernatant was loaded onto a Ni-NTA-agarose column (Qiagen) or pull-down, sequentially washed with 30 bed volumes (V) of buffer A (10 mM Tris–HCl, pH 8.0, 50 mM NaH 2 PO4, 10 mM imidazole) twice, 30 V of buffer B (10 mM Tris–HCl, pH 6.3, 50 mM NaH 2 PO4, 10 mM imidazole) twice, and eluted with 250 mM imidazole, pH 8.0. For denaturing Ni-NTA pull-down, cells were washed with cold PBS and lysed in lysis buffer (50 mM NaH 2 PO4, 300 NaCl, 8 M urea, PH 8.0), and spun down and the supernatant was subjected to Ni-NTA pull-down. Sequentially beads were washed with buffer A (10 mM Tris–HCl, pH 8.0, 50 mM NaH 2 PO4, 10 mM imidazole) twice and then buffer B (10 mM Tris–HCl, pH 6.3, 50 mM NaH 2 PO4, 10 mM imidazole) twice, and finally eluted with 250 mM imidazole, pH 8.0. In vitro binding analysis GST-PPARγ fusion protein was immobilized on glutathione-agarose beads in buffer (25 mM HEPES (pH 7.5), 6 mM NaCl and 0.2% NP-40) for 30 min 4 °C, and then in vitro translated proteins (p65) were added and incubated for another 2 h. Adsorbates to glutathione-conjugated beads were analysed by western blot. Luciferase assay HEK293T cells were transfected with NFκB-luc and Ptk-RL, plus various plasmids or shRNA, respectively. HEK293T cells were transfected with PPRE3-luciferase reporter and Ptk-RL plus PPARγ or mutant plasmids as indicated. Cell lysates were assayed by using a dual luciferase reporter assay system (Promega). EMSA analysis EMSAs were performed using the Lightshift Chemiluminescent EMSA kit (Pierce) for the NFκB consensus oligonucleotide probe, forward: 5′-GATCGAGGGGACTTT-CCCTAGC-3′, reverse: 5′-GCTAGGGAAAGTCCCC-TCGATC-3′, with 5′ end labelled with biotin (Thermo Scientific Biopolymers). Binding reactions were made in a total volume of 20 μl by adding 10 μg of nuclear extracts to 20 fmol of probe in binding buffer (20 mM HEPES (pH 8.0); 50 mM NaCl; 1mM EDTA; 5% glycerol; 0.05 mg ml −1 poly [dI-dC] and 0.5 mM dithiothreitol). After incubation at room temperature for 30 min, the electromobility shift of the probe was assayed in 6% native PAGE. Animal treatment Male 8- to 10-week-old mice (20–25 g) were fed standard mice chow pellets and had access to tap water. Mice were given PBS or pioglitazone (20m g kg −1 per day) for 3 days by oral gavage and then injected intravenously with 2 μg murine TNF-α for 6 h. Colonic tissues were harvested and total RNA was isolated for real-time PCR analysis. Xenograft tumour model NU/NU nude mice were purchased from (Charles River, USA). HT-29 cells were transfected with Vector (pcDNA3), p65, p65+PPARγ or K28R+PPARγ. Cells were selected with G418 to develop stable expressing cell lines. Various stable expressing plasmids in HT-29 cells (4 × 10 5 ) were injected subcutaneously in nude mice and after 4 weeks, tumour volume was measured with a digital caliper. WT or PPARγ −/− MEF cells (4 × 10 5 ) were injected subcutaneously in nude mice and after 4 weeks tumour volume was measured with a digital caliper. In other studies, HT-29 cells (1 × 10 6 ) were injected subcutaneously in nude mice and given PIOG (20 mg kg −1 per day) for 3 weeks by oral gavage. Tumour volume=1/2(length × width 2 ). Quantitative real-time PCR Total RNA was isolated using RNeasy Mini kit (QIAGEN) and analysed by Real Time PCR with SyBr Green (QIAGEN). mRNA expression was normalized against actin. Fold change over control was determined according to the Ct method [37] . Statistical analysis Data are expressed as the mean±s.e.m. Statistical comparison was carried out with one-way analysis of variance and Dunnett’s test. Significance was defined as P <0.05. How to cite this article: Yongzhong Hou, et al . PPARγ is an E3 ligase that induces the degradation of NFκB/p65. Nat. Commun. 3:1300 doi: 10.1038/ncomms2270 (2012).